Reducing the metabolic burden of rRNA synthesis promotes healthy longevity inCaenorhabditis elegans 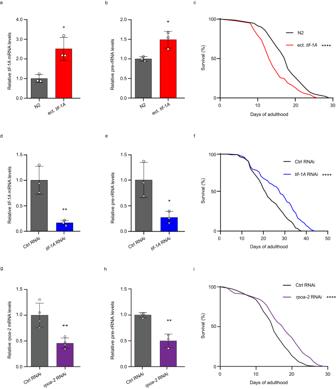Fig. 1: Attenuation of Pol I activity increases lifespan. a,bComparison oftif-1AmRNA (a) and pre-rRNA (b) levels inC. eleganswild-type (N2 Bristol) strain and COP2239 strain harboring an ectopictif-1Agene (ect.tif-1A). RT-qPCR data are shown relative to N2 and normalized totgb-1(tubulin gamma chain) mRNA. Each data point represents an independent biological sample ofn= 60 worms.cLifespan analysis of N2 and COP2239 (ect.tif-1A) strains,n= 140 worms.d,eRT-qPCR analysis oftif-1AmRNA (d) and pre-rRNA (e) levels in nematodes treated either with control (Ctrl) RNAi ortif-1ARNAi. Data are relative to Ctrl RNAi and normalized totgb-1mRNA. RNA from 3 independent experiments withn= 60 animals per sample was analyzed.fLifespan analysis of animals treated with Ctrl RNAi ortif-1ARNAi,n= 140 worms.g,hRelative levels ofrpoa-2mRNA (g) and pre-rRNA (h) in nematodes exposed to control (Ctrl) orrpoa-2RNAi. Samples from 4 (g) or 3 (h) biological replicates (n= 60 animals per sample) were used.iLifespan analysis of worms treated with Ctrl RNAi orrpoa-2RNAi,n= 140 worms. Fora,b,d,e,gandhdata represent mean values ± S.D.Pvalues were determined using a Student’s unpairedt-test. For lifespan analyses inc,fandi, results representative of 3 independent experiments are shown. Survival was scored daily.Pvalues were calculated using the Mantel-Cox test. ****P< 0.0001, **P< 0.01 and *P< 0.05. All statistical tests used were two-sided, the exactPvalues and statistical analyses are reported in the Source Data file.C. elegansculturing temperatures and RNAi treatment durations for this and other figures are provided in Supplementary Data23. Ribosome biogenesis is initiated by RNA polymerase I (Pol I)-mediated synthesis of pre-ribosomal RNA (pre-rRNA). Pol I activity was previously linked to longevity, but the underlying mechanisms were not studied beyond effects on nucleolar structure and protein translation. Here we use multi-omics and functional tests to show that curtailment of Pol I activity remodels the lipidome and preserves mitochondrial function to promote longevity in Caenorhabditis elegans . Reduced pre-rRNA synthesis improves energy homeostasis and metabolic plasticity also in human primary cells. Conversely, the enhancement of pre-rRNA synthesis boosts growth and neuromuscular performance of young nematodes at the cost of accelerated metabolic decline, mitochondrial stress and premature aging. Moreover, restriction of Pol I activity extends lifespan more potently than direct repression of protein synthesis, and confers geroprotection even when initiated late in life, showcasing this intervention as an effective longevity and metabolic health treatment not limited by aging. Aging is evolutionarily conserved, and four central nutrient-sensing pathways modulate healthspan and lifespan across taxa. The insulin/insulin-like growth factor signaling (IIS) and the mechanistic target of rapamycin (mTOR) promote anabolic reactions upon nutrient availability, whereas in a fasted state the adenosine monophosphate-activated protein kinase (AMPK) and the sirtuin family of nicotinamide adenine dinucleotide (NAD + )-dependent protein deacetylases trigger catabolic processes [1] , [2] . Shifting the balance from IIS and mTOR signaling towards AMPK and sirtuin activity by diverse interventions promotes longevity [1] , [2] . The IIS, mTOR, AMPK and sirtuin pathways impinge on Pol I-mediated transcription of rRNA genes (rDNA) into pre-rRNA, a precursor transcript comprising the three largest rRNAs [3] . Notably, Pol I activity accounts for the major part of cells’ transcription and, together with pre-rRNA processing and synthesis of ribosomal proteins, consumes a large portion of the cellular biosynthetic and energetic capacity [4] , [5] . Moreover, ribosome biogenesis is required for mRNA translation, placing pre-rRNA synthesis at the origin of the most energy-demanding cellular activities [4] , [6] . Two recent studies reported that perturbation of rRNA synthesis entails pro-longevity effects in C. elegans and D. melanogaster , either by inducing structural changes in the nucleolus, the organelle implicated in ribosome biogenesis, or by limiting protein synthesis, respectively [7] , [8] . However, the interplay between metabolic costs of Pol I activity and aging has not been explored in these studies. To link Pol I activity to cellular nutrient states, IIS, mTOR, and AMPK pathways target the essential Pol I transcription initiation factor 1A (TIF-1A, also known as TIF-IA or RRN3), which is conserved from yeast to human [9] . TIF-1A is inactivated by AMPK-mediated phosphorylation but requires IIS and mTOR-dependent phosphorylations to recruit Pol I to the rDNA promoter [10] , [11] , [12] . Thus, pre-rRNA synthesis and TIF-1A activity are likely to connect nutrient-sensing signaling and longevity regulation. Dietary restriction (DR) slows down aging across model organisms from yeast to non-human primates by redirecting cellular energy utilization from biosynthesis towards maintenance and repair [2] . Notably, DR and DR-mimetic drugs like metformin were recently found to lose their geroprotective efficacy in late life due to aging-associated decline of metabolic plasticity [13] , [14] . Thus, novel pro-longevity compounds and interventions without age restriction are needed. In this study, we identified an anti-correlation between rDNA transcription and longevity. Using genetics, omics, and functional assays in Caenorhabditis elegans and human primary fibroblasts, we showed that curtailment of pre-rRNA synthesis not only inhibits translation but also moderates energy expenditure and supports metabolic health during aging. The geroprotective efficacy of Pol I restriction does not decline with age, demonstrating its possible late-in-life use as a lifespan and healthspan extension treatment. Levels of pre-rRNA synthesis control lifespan and healthspan To increase TIF-1A levels (encoded by the tif-1A/C36E8.1 gene in C. elegans ), we generated a strain harboring the C36E8.1 cDNA fused to a Ty1-epitope tag (Supplementary Figs. 1a and 17a, b ). Reverse transcription followed by quantitative PCR (RT-qPCR) revealed a ~2.5-fold increase in total tif-1A mRNA levels, in turn elevating pre-rRNA levels by ~1.5-fold (Fig. 1a, b ). Notably, tif-1A overexpression conferred lifespan shortening, indicating that enhanced pre-rRNA synthesis accelerates aging in nematodes (Fig. 1c ). To test if restraining rDNA activity has the opposite effect, we used RNA interference (RNAi)-mediated gene knockdown (KD) to reduce tif-1A expression. Compared with the non-targeting RNAi control, both tif-1A mRNA and pre-rRNA levels were efficiently diminished when worms were reared for two generations on double-stranded RNA (dsRNA) producing bacteria (Fig. 1d, e ). In addition, we observed that the tif-1A KD reduced nucleolar size (Supplementary Fig. 1b, c ), a trait that correlates with ribosomal biogenesis and is linked to longevity [7] , [8] . Accordingly, the lifespan of TIF-1A-depleted worms was extended by approximately 30% (Fig. 1f ). To further confirm life extension through reduced Pol I activity, we used RNAi against rpoa-2 , encoding the second largest Pol I subunit [15] . When initiated in L4 larvae, the rpoa-2 KD was efficient after two days, eliciting a reduction in rpoa-2 mRNA as well as pre-rRNA levels (Fig. 1g, h ). In accord with the tif-1A KD phenotype, rpoa-2 RNAi significantly extended lifespan (Fig. 1i ), corroborating the geroprotective effect of restricted pre-rRNA synthesis in adult animals. Fig. 1: Attenuation of Pol I activity increases lifespan. a , b Comparison of tif-1A mRNA ( a ) and pre-rRNA ( b ) levels in C. elegans wild-type (N2 Bristol) strain and COP2239 strain harboring an ectopic tif-1A gene (ect. tif-1A ). RT-qPCR data are shown relative to N2 and normalized to tgb-1 (tubulin gamma chain) mRNA. Each data point represents an independent biological sample of n = 60 worms. c Lifespan analysis of N2 and COP2239 (ect. tif-1A ) strains, n = 140 worms. d , e RT-qPCR analysis of tif-1A mRNA ( d ) and pre-rRNA ( e ) levels in nematodes treated either with control (Ctrl) RNAi or tif-1A RNAi. Data are relative to Ctrl RNAi and normalized to tgb-1 mRNA. RNA from 3 independent experiments with n = 60 animals per sample was analyzed. f Lifespan analysis of animals treated with Ctrl RNAi or tif-1A RNAi, n = 140 worms. g , h Relative levels of rpoa-2 mRNA ( g ) and pre-rRNA ( h ) in nematodes exposed to control (Ctrl) or rpoa-2 RNAi. Samples from 4 ( g ) or 3 ( h ) biological replicates ( n = 60 animals per sample) were used. i Lifespan analysis of worms treated with Ctrl RNAi or rpoa-2 RNAi, n = 140 worms. For a , b , d , e , g and h data represent mean values ± S.D. P values were determined using a Student’s unpaired t -test. For lifespan analyses in c , f and i , results representative of 3 independent experiments are shown. Survival was scored daily. P values were calculated using the Mantel-Cox test. **** P < 0.0001, ** P < 0.01 and * P < 0.05. All statistical tests used were two-sided, the exact P values and statistical analyses are reported in the Source Data file. C. elegans culturing temperatures and RNAi treatment durations for this and other figures are provided in Supplementary Data 23 . Full size image In C. elegans , the RNA-binding protein NCL-1 inhibits pre-rRNA processing and in turn ribosome biogenesis by downregulating the rRNA 2’-O-methyltransferase fibrillarin/FIB-1 [16] . We found that NCL-1 also dampens pre-rRNA synthesis, RNA-mediated KD of ncl-1 elevating pre-rRNA levels and, in line with previous work [8] , shortening lifespan (Fig. 2a–c ). Thus, ncl-1 RNAi had similar molecular and physiological effects as tif-1A overexpression, and both manipulations contrasted the effects of tif-1A and rpoa-2 KDs. Fig. 2: Pre-rRNA expression is inversely correlated with lifespan and healthspan. a , b RT-qPCR analysis of ncl-1 mRNA ( a ) and pre-rRNA ( b ) levels of worms treated either with control (Ctrl) RNAi or ncl-1 RNAi. Values are relative to Ctrl RNAi and normalized to tgb-1 mRNA. Mean ± S.D. values of 3 independent experiments ( n = 60 worms per sample) are shown. c Lifespan analysis of the nematodes upon treatment with Ctrl RNAi or ncl-1 RNAi, n = 140 worms. Survival was scored daily and P values were calculated using the Mantel-Cox test. Result is representative of 3 independent trials. d Body size (area) measurement of animals treated with Ctrl, tif-1A or ncl-1 RNAi. n = 30 worms. Data combine three independent trials and mean ± S.D. is shown. e Schematic of the locomotor performance test (burrowing assay). f , g Burrowing assays of animals treated with Ctrl, tif-1A or ncl-1 RNAi. The % of animals reaching the surface was determined at the indicated time points. Data show mean values ± S.D. of 3 independent assays performed on the second day of adulthood (AD2) with n = 40–45 worms ( f ) or on AD12 with n = 40–60 worms ( g ). P values were calculated with the Mantel-Cox test. h , i Representative images ( n = 10 worms per image) and quantification of intestinal integrity monitored by the Brilliant Blue dye retention assay. Worms with staining outside the gut (‘Smurf’ phenotype) were scored following treatment with Ctrl, tif-1A or ncl-1 RNAi ( n = 40–60 worms per treatment) at AD2 ( h ) or AD12 ( i ), scale bar 200 μm. Mean ± S.D. values of 3 independent experiments are shown. P values were determined using a Student’s unpaired t -test. ns = not significant, **** P < 0.0001, *** P < 0.001, ** P < 0.01, * P < 0.05. All statistical tests used were two-sided, the exact P values and statistical analyses are reported in the Source Data file. Full size image Measurement of body size revealed that on the second day of adulthood (AD2, young adult animals), ncl-1 KD worms were bigger than the control animals, whereas TIF-1A-depleted worms were significantly smaller (Fig. 2d ). At old age (AD12), body size was increased and equalized across treatment groups (Fig. 2d ), suggesting that tif-1A RNAi worms gained on the other two groups with age. We next carried out a neuromuscular performance (NMP) test monitoring the ability of worms to burrow through a pluronic gel towards bacteria applied on the top [17] (Fig. 2e ). At AD2, the NMP correlated with the extent of rRNA gene transcription, i.e., NCL-1 and TIF-1A depletion conferred superior and inferior neuromuscular fitness, respectively (Fig. 2f ). However, the fitness of TIF-1A-depleted nematodes remained stable throughout life while the performance of control animals, and even more so of the ncl-1 RNAi group, declined, rendering tif-1A KD worms the fittest at AD12 (Fig. 2g ). Given the observed fitness differences, we next assessed intestinal integrity as another health parameter associated with longevity [18] . We fed worms with Brilliant Blue, which only exits the intestine when its barrier function is compromised, causing whole body staining (‘Smurf’ phenotype) [19] . While barely detectable at young age, Smurf formation increased at AD12, being the highest upon NCL-1 depletion (~80%) and lowest in TIF-1A-deficient worms (~40%) (Fig. 2h, i ). Notably, a previous study in D. melanogaster also connected reduced Pol I activity with improved intestinal integrity at old age [7] , demonstrating the evolutionary conservation of this phenomenon. These findings show that elevation of pre-rRNA synthesis confers a fitness advantage early in life but accelerates health decline with age, while its restriction limits early life fitness transiently and eventually prolongs both lifespan and healthspan. rDNA activity modulates ribosome biogenesis and metabolism To address the mechanisms causing inverse correlation between pre-rRNA levels and longevity, worms treated with control, tif-1A, and ncl-1 RNAi were collected at AD2, AD6, and AD12 (young, middle and old age, respectively), and proteomes were profiled by mass-spectrometry detecting ∼ 5000 proteins in each sample (Supplementary Fig. 2 ). Principal component analysis (PCA) revealed differences between the age groups and RNAi treatments, with tif-1A KD animals clustering apart from controls at all ages, while ncl-1 KD exhibited some overlap with controls (Supplementary Fig. 3 ). Notably, the two KDs shifted from controls in opposite directions, underscoring their different effects on lifespan. We next performed pairwise comparisons either of AD12 versus AD2 in the control RNAi group, or of tif-1A and ncl-1 RNAi versus control RNAi at AD2, 6, and 12, thereby monitoring age- or rDNA activity-dependent proteome remodeling, respectively (Supplementary Data 1 ). In the initial targeted analysis, we focused on markers of adaptive stress responses previously linked to longevity, i.e., immune response (C-type lectins; CLECs), heat stress response (heat shock proteins; HSPs), and oxidative stress response (glutathione-S-transferases; GSTs) [14] . While the expression of several individual markers was significantly changed, we found that tif-1A RNAi treatment did not lead to an overall modulation of these three responses (Fig. 3a and Supplementary Data 2 ). Similarly, ncl-1 KD worms showed no global changes in CLECs and HSPs but had persistently low expression of GSTs, indicating alterations in redox balance, which could impact mitochondrial homeostasis [20] (Fig. 3b and Supplementary Data 3 ). In contrast to the stress response pathways, ribosomal proteins and the lipid droplet-associated vitellogenins (VITs) [21] , [22] were strongly reduced by tif-1A KD (Fig. 3a and Supplementary Data 2 ), whereas in ncl-1 RNAi exposed nematodes, the downregulation of VITs was less pronounced and ribosomal content became moderately upregulated with age (Fig. 3b and Supplementary Data 3 ). Fig. 3: Proteomics links Pol I activity, ribosomal content and metabolism. a – f Proteomes of nematodes treated with control (Ctrl) RNAi, tif-1A RNAi or ncl-1 RNAi were analyzed at AD2, AD6 and AD12. Each condition has five biological replicates of n = 700 worms. a , b Box plots showing log2 fold changes of selected immune response (CLEC), heat stress response (HSP), oxidative stress response (GST), and ribosomal (Ribosome) proteins as well as vitellogenins (VIT), comparing tif-1A KD ( a ) and ncl-1 KD ( b ) nematodes to age-matched controls. Each dot represents one protein, the median fold change within each group is shown as a bold line, the lower and upper limits of the boxplot indicate the first and third quartile, respectively, and the whiskers show the most up- and down-regulated proteins. The expression levels and Q values of individual proteins are reported in Supplementary Data 1 – 3 . c , d Proteins differentially expressed (log2 fold change > 0.58, Q value < 0.05) in tif-1A KD ( c ) and ncl-1 KD ( d ) versus Ctrl RNAi animals on AD12 were classified using WormCat, and the two top enriched categories (Ribosome and Metabolism) with their subgroups are presented (analysis details are shown in Supplementary Data 8 and 9 ). e Box plots showing log2 fold changes of selected mitochondrial proteins between AD2 and AD12 Ctrl RNAi animals are presented. Either all measured mitochondrial proteins (‘mitochondrion’) or distinct categories (‘mito-protein complex’, ‘mito-respirasome’ and (‘mito-translation’) are shown. f Box plots showing log2 fold changes of selected mito-ribosome components in tif-1A RNAi and ncl-1 RNAi worms compared to age-matched controls. The expression levels and Q values of individual proteins are reported in Supplementary Data 10 (for e ) and 11 (for f ). In a , b , e and f the Wilcoxon rank-sum test was used for statistical analysis; Bonferroni correction was performed to adjust for multiple comparisons. ns = not significant, **** P < 0.0001, *** P < 0.001, ** P < 0.01, * P < 0.05. All statistical tests used were two-sided, the exact P values and statistical analyses are reported in the Source Data file. Full size image To assess the data by an additional unbiased method, the WormCat tool [23] was used to categorize proteins differentially expressed between old control and tif-1A RNAi or ncl-1 RNAi worms (Supplementary Data 4 – 9 ). Ribosome and metabolism were indeed the two top enriched categories, (Supplementary Figs. 4 and 5 ; Supplementary Data 5 and 7 ), metabolism even surpassing ribosomal processes in the proportion of regulated proteins in both KDs (Fig. 3c, d ; Supplementary Data 8 and 9 ). While changes in ribosomal biogenesis in animals harboring differential rDNA output were expected [7] , [8] , the strong prevalence of changes in lipid and mitochondrial metabolism was unexpected and warranted further investigation. Previous studies have reported that the abundance of mitochondrial proteins, including components of the mitochondrial ribosome (mito-ribosome), decreases with age [24] , which in turn functionally impacts longevity [14] . Accordingly, our analysis of control animals during aging confirmed these findings (Fig. 3e and Supplementary Data 10 ). Interestingly, mito-ribosomal content, which correlates with mitochondrial abundance, was differentially regulated by tif-1A and ncl-1 RNAi, with ncl-1 KD causing a strong increase in the abundance of mito-ribosomal proteins throughout life, and tif-1A KD promoting a moderate but significant elevation of mito-ribosomal protein levels with the biggest effect seen at old age (AD12) (Fig. 3f and Supplementary Data 11 ). This result suggested that rDNA activity impacts organismal fitness and longevity by modulating mitochondrial homeostasis. Curbed ribosome biogenesis delays metabolic aging The persistently low abundance of ribosomal proteins in tif-1A RNAi animals (Fig. 3a ) was paralleled by downregulation of total protein levels (Supplementary Fig. 6a ). In line with the previously shown reduction of protein synthesis in long-lived flies with partially impaired Pol I function [7] , this finding suggested that dampening of translation might contribute to life extension caused by tif-1A RNAi. In fact, reducing the translational output can counteract the loss of proteostasis, which is a hallmark of aging [25] . To elucidate to which extent tif-1A deficiency promotes longevity via translation inhibition, we combined tif-1A knockdown with the life-extending impairment of the ife-2 gene encoding an isoform of the eukaryotic translation initiation factor 4E (eIF-4E) [26] . Lifespans of wild-type and ife-2 mutant worms treated with either control or tif-1A RNAis, were assessed. Upon control treatment, the ife-2 mutants lived moderately longer than wild-type animals, while tif-1A RNAi prolonged lifespan in both strains to similar levels (Fig. 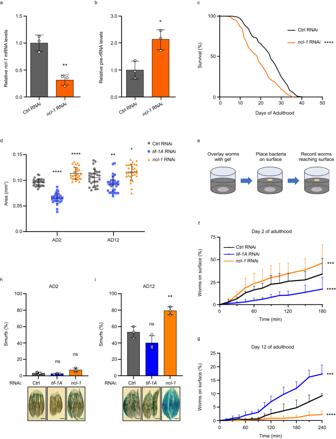Fig. 2: Pre-rRNA expression is inversely correlated with lifespan and healthspan. a,bRT-qPCR analysis ofncl-1mRNA (a) and pre-rRNA (b) levels of worms treated either with control (Ctrl) RNAi orncl-1RNAi. Values are relative to Ctrl RNAi and normalized totgb-1mRNA. Mean ± S.D. values of 3 independent experiments (n= 60 worms per sample) are shown.cLifespan analysis of the nematodes upon treatment with Ctrl RNAi orncl-1RNAi,n= 140 worms. Survival was scored daily andPvalues were calculated using the Mantel-Cox test. Result is representative of 3 independent trials.dBody size (area) measurement of animals treated with Ctrl,tif-1Aorncl-1RNAi.n= 30 worms. Data combine three independent trials and mean ± S.D. is shown.eSchematic of the locomotor performance test (burrowing assay).f,gBurrowing assays of animals treated with Ctrl,tif-1Aorncl-1RNAi. The % of animals reaching the surface was determined at the indicated time points. Data show mean values ± S.D. of 3 independent assays performed on the second day of adulthood (AD2) withn= 40–45 worms (f) or on AD12 withn= 40–60 worms (g).Pvalues were calculated with the Mantel-Cox test.h,iRepresentative images (n= 10 worms per image) and quantification of intestinal integrity monitored by the Brilliant Blue dye retention assay. Worms with staining outside the gut (‘Smurf’ phenotype) were scored following treatment with Ctrl,tif-1Aorncl-1RNAi (n= 40–60 worms per treatment) at AD2 (h) or AD12 (i), scale bar 200 μm. Mean ± S.D. values of 3 independent experiments are shown.Pvalues were determined using a Student’s unpairedt-test. ns = not significant, ****P< 0.0001, ***P< 0.001, **P< 0.01, *P< 0.05. All statistical tests used were two-sided, the exactPvalues and statistical analyses are reported in the Source Data file. 4a ). When we impeded translation elongation with cycloheximide (CHX), which also extends the lifespan of C. elegans [27] , tif-1A RNAi was again more potent, increasing survival of worms similarly in the absence or presence of CHX (Supplementary Fig. 6b ). These results indicate that the effects of tif-1A knockdown surpass those of translational inhibition by CHX or ife-2 mutation with respect to lifespan extension. It cannot, however, be excluded that tif-1A KD reduces translation more potently. Fig. 4: Pol I inhibition decelerates metabolic aging. a Survival analysis of C. elegans wild-type (N2 Bristol) and ife-2 mutant strains treated with control (Ctrl) RNAi or tif-1A RNAi, n = 140 worms. b Comparison of ATP pools at AD2 between wild-type (N2) and ife-2 mutant worms treated with Ctrl RNAi or tif-1A RNAi. ATP levels were measured in a bioluminescence assay and normalized to total protein content. Values are shown relative to N2 Ctrl RNAi. Data are from 6 independent experiments with n = 50 worms in each sample. Mean ± S.D. values are shown. c Comparison of ATP pools at AD2 and AD12 between worms treated with Ctrl RNAi or tif-1A RNAi. ATP measurement was conducted as in b , and values are relative to Ctrl RNAi on AD12. Mean ± S.D. values of 6 independent experiments with n = 50 worms are shown. d Survival analysis of worms exposed to Ctrl RNAi or tif-1A RNAi and, from AD12 onwards, to 50 mM metformin (Met), n = 140 animals. A representative result of four independent experiments is shown. For a and d , survival was scored daily and P values were determined using the Mantel-Cox test. For b and c , a Student’s unpaired t -test was used for statistics. e , f BJ primary human skin fibroblasts were treated with indicated doses of metformin in the absence (DMSO) or presence of the indicated concentrations of ATP (positive survival control) or the Pol I inhibitors BMH-21 ( e ) and CX-5461 ( f ). Mitochondrial activity was assessed by MTT assay, and an unpaired Student’s t -test was used to compute P values, comparing each co-treatment to the respective DMSO + Metformin control condition, data represent mean ± S.D of 3 independent experiments. ns = not significant, **** P < 0.0001, *** P < 0.001, ** P < 0.01, * P < 0.05. All statistical tests used were two-sided, the exact P values and statistical analyses are reported in the Source Data file. Full size image Subsequently, we explored the connection between rDNA activity, protein synthesis, and energy metabolism, because rDNA transcription is not only a prerequisite for protein synthesis, but also initiates highly energy-demanding pre-rRNA processing and ribosome assembly [4] , [5] . Accordingly, we observed a ~1.5-fold elevation of adenosine triphosphate (ATP) content in TIF-1A-depleted worms relative to control animals (Fig. 4b ). Notably, ife-2 mutant worms and wild-type animals exhibited similar baseline ATP levels and showed comparably elevated ATP content upon tif-1A RNAi treatment (Fig. 4b ), indicating that restriction of pre-rRNA synthesis may override translational repression in terms of cellular energy conservation. The possible difference in the extent of translational inhibition between ife-2 mutation and tif-1A RNAi treatment could also be contributing. Given the tight cross-regulation between synthesis of pre-rRNA and ribosomal proteins [28] , [29] , we wondered whether depletion of the ribosomal protein RPS-15, which was previously reported to extend lifespan in C. elegans [30] , elicits energy saving similar to tif-1A KD. In fact, rps-15 RNAi treatment increased whole organism ATP levels, suggesting that perturbation of various steps of ribosome biogenesis reduces energy expenditure and prolongs lifespan (Supplementary Fig. 6c ). Aging-associated reduction of the cellular ATP pool has been observed in C. elegans and other animals contributing to the aging-associated metabolic decline [31] . Importantly, tif-1A KD was effective in counteracting this trait, and it boosted the ATP content in old KD worms (AD12) to levels comparable to young control animals (AD2) (Fig. 4c ). It was recently shown that mitochondrial inhibitor metformin causes ATP exhaustion and toxicity in aged nematodes due to deterioration of their mitochondria [14] . As tif-1A depletion preserved both the mito-ribosome levels and the ATP content in late life (Figs. 3f and 4c ), we tested whether it improved the metabolic resilience at old age by using metformin toxicity as a proxy readout [14] . In control animals, metformin administration from AD12 onwards induced the expected lethality and most animals died within 72 hours (Fig. 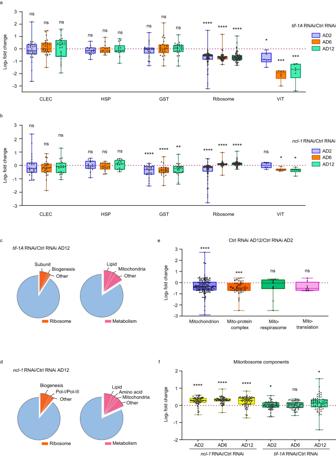Fig. 3: Proteomics links Pol I activity, ribosomal content and metabolism. a–fProteomes of nematodes treated with control (Ctrl) RNAi,tif-1ARNAi orncl-1RNAi were analyzed at AD2, AD6 and AD12. Each condition has five biological replicates ofn= 700 worms.a,bBox plots showing log2 fold changes of selected immune response (CLEC), heat stress response (HSP), oxidative stress response (GST), and ribosomal (Ribosome) proteins as well as vitellogenins (VIT), comparingtif-1AKD (a) andncl-1KD (b) nematodes to age-matched controls. Each dot represents one protein, the median fold change within each group is shown as a bold line, the lower and upper limits of the boxplot indicate the first and third quartile, respectively, and the whiskers show the most up- and down-regulated proteins. The expression levels and Q values of individual proteins are reported in Supplementary Data1–3.c,dProteins differentially expressed (log2 fold change > 0.58, Q value < 0.05) intif-1AKD (c) andncl-1KD (d) versus Ctrl RNAi animals on AD12 were classified using WormCat, and the two top enriched categories (Ribosome and Metabolism) with their subgroups are presented (analysis details are shown in Supplementary Data8and9).eBox plots showing log2 fold changes of selected mitochondrial proteins between AD2 and AD12 Ctrl RNAi animals are presented. Either all measured mitochondrial proteins (‘mitochondrion’) or distinct categories (‘mito-protein complex’, ‘mito-respirasome’ and (‘mito-translation’) are shown.fBox plots showing log2 fold changes of selected mito-ribosome components intif-1ARNAi andncl-1RNAi worms compared to age-matched controls. The expression levels and Q values of individual proteins are reported in Supplementary Data10(fore) and 11 (forf). Ina,b,eandfthe Wilcoxon rank-sum test was used for statistical analysis; Bonferroni correction was performed to adjust for multiple comparisons. ns = not significant, ****P< 0.0001, ***P< 0.001, **P< 0.01, *P< 0.05. All statistical tests used were two-sided, the exactPvalues and statistical analyses are reported in the Source Data file. 4d ). In contrast, tif-1A -deficient worms survived much longer in the presence of metformin, although their median lifespan was also reduced relative to the untreated control (Fig. 4d ). This result indicated that restriction of rRNA synthesis sustains energy metabolism and metabolic plasticity during aging in C. elegans . Finally, we investigated if pharmacological inhibition of pre-rRNA synthesis can stabilize cellular energy metabolism similar to the genetic disruption of Pol I activity. We used metformin treatment to induce aging-like metabolic stress in human primary fibroblasts [14] , and combined metformin exposure with Pol I inhibition by the compounds BMH-21 and CX-5461 [32] , [33] , with direct ATP repletion serving as a positive control. In accord with previous data [34] , both inhibitors caused a dose-dependent decline of pre-rRNA levels (Supplementary Fig. 7a, b ) as well as increased expression of the senescence marker p21 (Supplementary Fig. 7c, d ). Consistent with the previously reported slowing of cellular growth and proliferation by Pol I inhibitors [34] , [35] , BMH-21 and CX-5461 elicited a slight reduction of baseline mitochondrial activity as measured by the MTT assay, while strong ablation of mitochondrial function by metformin was alleviated by both drugs (Fig. 4e, f ). These results demonstrated that stabilization of energy homeostasis and mitochondrial function by the reduction of rDNA activity is conserved between nematodes and humans, and can be achieved by pharmaceuticals. However, as both BMH-21 and CX-5461 induce cellular senescence, they are not suited for life-extension drugs. In addition, metformin treatment potentiates the cytotoxic effects of the CX-5461 in a murine lymphoma model [36] . This phenomenon is likely driven by specific alterations of cancer cell metabolism but it speaks against the possible co-administration of both drugs in the clinic. rDNA activity contributes to lipidome changes in aging Metformin toxicity has been linked not only to mitochondrial homeostasis but also to alterations in lipid metabolism [14] , [37] . As lipid metabolism was highlighted in the proteomics profiles of Pol I-modulated animals (Fig. 3c, d ), we analyzed the lipidomes of control, tif-1A KD and ncl-1 KD worms on AD2, AD6, and AD12. We found that in control animals fed with an HT115 E. coli diet, the levels of phosphatidylcholines (PCs), phosphatidylethanolamines (PEs), and phosphatidylserines (PSs) increased between young and middle age and remained elevated also later in life (Fig. 5a and Supplementary Data 12 ). Interestingly, the aging-linked increase in phospholipids was abrogated in tif-1A KD worms, while ncl-1 KD animals demonstrated their premature elevation on AD2, followed by an accelerated exhaustion on AD12 (Fig. 5a ), revealing differential lipidome trajectories between the two KDs. Fig. 5: Pol I activity affects the lipidome and mitochondria. a Lipid abundance in control (Ctrl) RNAi, tif-1A RNAi and ncl-1 RNAi animals at different ages, normalized to the internal standard and animal number ( n = 700). Values were computed from absolute intensities; mean of 5 biological replicates expressed as % of Ctrl RNAi treatment at AD2 is shown in each case (see Supplementary Data 12 for raw data). PC phosphatidylcholine, PE phosphatidylethanolamine, PS phosphatidylserine, PI phosphatidylinositol, PG phosphatidylglycerol, TAG triacylglycerol, FFA free fatty acid. b Volcano plots of lipid species separated by age (AD 2, 6, 12) and fatty acid desaturation. SFA saturated fatty acid, MUFA monounsaturated fatty acid, PUFA polyunsaturated fatty acid. Horizontal axis subtracts Ctrl RNAi mean log 10 values from respective tif-1A RNAi (left panel) or ncl-1 RNAi (right panel) values for each lipid, with statistics performed by multiple unpaired t -test on log-transformed mean values using a two-stage linear step-up procedure by Benjamini, Krieger and Yekutieli, FDR = 5%, data are from 5 biological replicates with n = 700 worms each. Calculations (from relative intensities) are shown in Supplementary Data 13 – 15 . c Ratio of MUFAs to PUFAs in PCs at indicated age upon treatment with Ctrl RNAi, tif-1A RNAi or ncl-1 RNAi. Mean ± S.D. values from 5 replicates each with n = 700 worms are shown. Calculations (from relative intensities) are shown in Supplementary Data 19 . d Fluorescence measurements in nematodes expressing hsp-6p::GFP following exposure to Ctrl, mip-1 , ncl-1 or tif-1A RNAi. mip-1 RNAi served as a positive mito-stress control. n = 20-25 worms per condition. Representative result of 3 independent trials. For c and d , Student’s unpaired t -test compared ncl-1 and tif-1A RNAi effects to the age-matched Ctrl RNAi baseline. e – g Survival analysis of wild-type (N2 Bristol strain) and atfs-1 (gk3094) mutant nematodes ( e ), or N2 worms treated from AD1 onwards with the vehicle DMSO or 25 µM FCCP ( f ), or N2 and skn-1 (zj15) mutant nematodes ( g ), exposed to Ctrl or rpoa-2 RNAi, survival was scored daily. Representative results of three independent experiments, n = 140 worms, statistics assessed by Mantel-Cox test. ns = not significant, **** P < 0.0001, *** P < 0.001, ** P < 0.01, * P < 0.05. All statistical tests used were two-sided, the exact P values and statistical analyses are reported in the Source Data file. Full size image We next examined the lipidomes of tif-1A and ncl-1 KD nematodes for features that were previously linked to increased longevity, i.e., elevated levels of monounsaturated fatty acids (MUFAs) as well as reduced levels of oxidative damage-prone polyunsaturated FAs (PUFAs) and lipotoxicity-associated saturated FAs (SFAs) [38] , [39] , [40] . This pattern was indeed observed in long-lived tif-1A KD animals across age points and lipid classes, while ncl-1 KD showed an opposite trend consistent with the shortened lifespan of these animals (Fig. 5b and Supplementary Fig. 8a ; Supplementary Data 13 – 16 ). In addition, the analysis of the relative phospholipid proportions showed different trends between the two KDs: the percentages of PCs and PSs were elevated and the fractions of PEs and PGs were reduced in aged tif-1A KD worms, while opposite changes were seen upon ncl-1 KD (Supplementary Fig. 8b–g and Supplementary Data 17 ). Notably, a higher PC/PE ratio has previously been linked to extended longevity as PCs are less prone to oxidative damage compared to PEs [38] . At the level of distinct lipid classes, an increase of the MUFA/PUFA ratio was observed in tif-1A KD animals, with particular significance seen for PCs and PEs (Fig. 5c , Supplementary Fig. 9a, b and Supplementary Data 18 , 19 ). As MUFAs are less susceptible to peroxidation, a high MUFA/PUFA ratio entails pro-longevity effects [39] , [40] . Contrary to the effect of tif-1A RNAi, the ncl-1 RNAi administration caused a premature decline of MUFA content across lipid types (Fig. 5c , Supplementary Fig. 9a, b and Supplementary Data 18 , 19 ). In addition, the relative levels of SFAs in distinct lipid types showed trends of elevation in ncl-1 KD animals and this trend was inverted in tif-1A inactivated worms (Supplementary Fig. 9c and Supplementary Data 18 ), again consistent with opposite effects on longevity of the two KDs. Finally, we assessed specific triacylglyceride (TAG) features that were previously identified as markers of metabolic aging and mitochondrial dysfunction, i.e., increased FA chain length and number of double bonds higher than three ( n ≥ 3 PUFAs) [40] . Importantly, both features were reduced by tif-1A RNAi treatment, and they were prematurely increased in ncl-1 KD animals (Supplementary Fig. 10a, b and Supplementary Data 19 ). Collectively, the lipidomics profile of tif-1A KD was consistent with attenuated aging while ncl-1 KD animals showed elevated levels of lipids that are prone to oxidative damage (such as PUFA-containing PEs) and enrichment in signatures previously associated with aging-induced mitochondrial dysfunction. Pol I transcription promotes mitochondrial stress To test the link between rDNA transcription and mitochondrial stress, we examined GFP expression in young animals harboring a reporter ( hsp-6p::GFP ) for the stress-induced mitochondrial chaperone gene hsp-6 [41] exposed to non-targeting, tif-1A , or ncl-1 RNAi. We found that increasing pre-rRNA synthesis by ncl-1 RNAi exacerbated mitochondrial stress, while stress was alleviated by the Pol I-constraining tif-1A RNAi (Fig. 5d and Supplementary Fig. 11 ). Mitochondrial stress in young ncl-1 KD animals was corroborated by elevated proportions of fragmented and very fragmented mitochondria (Supplementary Fig. 12a, b )—a phenotype associated with metabolic aging [14] , [42] . Interestingly, we observed a modest elevation of mitochondrial fission upon reduction of Pol I activity (Supplementary Fig. 12a, b ), prompting us to investigate the link between remodeling of mitochondria, rRNA synthesis, and longevity. Nematodes deficient in either mitochondrial fusion ( fzo-1 mutant) or fission ( drp-1 mutant) [43] were not hampered in lifespan extension upon exposure to rpoa-2 RNAi, demonstrating that mitochondrial remodeling is not relevant for the crosstalk between rDNA and lifespan (Supplementary Fig. 12c, d ). To test if perturbation of Pol I triggers mitochondrial stress responses, we knocked down rpoa-2 in worm strains lacking key regulators of either the mitochondrial unfolded protein response (UPR mt ) ( atfs-1 ) [44] or mitophagy (pink-1 ) [45] , but observed the same relative lifespan extension by rpoa-2 RNAi in wild-type and mutant animals (Fig. 5e and Supplementary Fig. 13a ). Concurrently, our lipidomic profiling revealed enrichment of the stress-limiting lipokine PI(18:1/18:1) [46] by tif-1A KD, especially in old worms, while it was depleted by ncl-1 KD throughout life (Supplementary Fig. 13b and Supplementary Data 20 ). Although a direct influence of PI(18:1/18:1) on mitochondria has not been shown, its pleiotropic effect on several cellular stress responses [46] may contribute to differential mitochondrial health of the KD animals. To further test the role of mitochondrial integrity in life extension by lowered rDNA activity, we combined rpoa-2 RNAi with the dose-dependent poisoning of mitochondria by the uncoupling agent FCCP [47] . Interestingly, the full longevity benefit of Pol I perturbation was maintained only at the lowest concentration of the drug, while higher FCCP doses diminished and even reversed the life extension of rpoa-2 KD animals (Fig. 5f and Supplementary Fig. 13c, d ). These findings confirm the key role of mitochondria in life extension by reduced Pol I activity and corroborate the ability of Pol I repression to buffer moderate mitochondrial stress, without involvement of UPR mt and mitophagy. Finally, we tested if longevity extension by reduced rDNA transcription engages a conserved transcription factor SKN-1/Nrf2 with known roles in protective mechanisms such as mitochondrial biogenesis [45] , oxidative stress response [48] , and lipid metabolism [38] . By combining rpoa-2 RNAi with a loss-of-function mutation of skn-1 , we found that Pol I restriction shortened the lifespan of skn-1 mutants contrary to the prolongation seen in wild-type controls (Fig. 5g ), demonstrating a functional link between rDNA transcription and SKN-1-mediated cellular responses including modulation of mitochondrial health. TAG turnover connects Pol I activity to mitochondrial stress We next explored the hierarchical relationship between mitochondria and lipid metabolism in mediating longevity benefits of reduced Pol I activity. As a starting point, we revisited the lipidome profiles of control, tif-1A KD, and ncl-1 KD animals at different ages (Fig. 5a ). Interestingly, we noticed that in the background of broadly reduced lipid content, the storage TAG levels were specifically elevated in tif-1A KD nematodes at old and middle age. Likewise, Oil Red O staining indicative of TAG levels [49] was increased in middle-aged rpoa-2 KD animals (Supplementary Fig. 14a ). In contrast, old and middle-aged ncl-1 KD animals showed accelerated exhaustion of TAGs (Fig. 5a ), indicating premature loss of the energy storage and revealing opposite regulation of TAG turnover between the two KDs, in line with their inverse longevity phenotypes. Importantly, the decline of TAGs, which reside in lipid droplets [22] , was accompanied by the moderate reduction of the protein lipid droplet components VITs in ncl-1 KD worms (Fig. 3b ). Conversely, the strong downregulation of VITs in tif-1A RNAi animals (Fig. 3a ) occurred amid stably high levels of TAGs, suggesting lipid droplet remodeling towards a higher lipid-to-protein ratio, which was previously linked to DR in facilitating effective regulation of TAG metabolism [50] . To test if TAG turnover is implicated in the differential longevity upon reduced or forced Pol I activity, we combined rpoa-2 RNAi or ncl-1 RNAi with knockdown of the atgl-1 gene, encoding the C. elegans orthologue of the adipose triglyceride lipase (ATGL). ATGL-1 is implicated in mobilization of TAGs [51] and regulates responses to differential nutrient availability during dauer diapause and fasting [52] , [53] . Strikingly, both life extension of rpoa-2 KD and lifespan reduction of ncl-1 KD were reversed by co-inactivation of atgl-1 (Fig. 6a, b ), revealing the involvement of TAG metabolism in the longevity effects of differential Pol I activity. At the same time, dampening of peroxisome activity by mutation of prx-5 , which encodes a peroxisome assembly factor [37] , [54] had no impact on life extension by lowered pre-rRNA synthesis (Fig. 6c ). Moreover, interference with mitochondrial fatty acid β-oxidation by RNAi against acs-2 [55] , and curbing of fatty acid desaturation by KD of the Δ9 desaturase fat-5 [39] , [56] did not affect the longevity benefits of reduced Pol I activity (Fig. 6d and Supplementary Fig. 14b–d ). This neutral behavior of both interventions occurred despite a clear upregulation of ACS-2 and FAT-5 proteins in old tif-1A KD animals (Supplementary Fig. 14e and Supplementary Data 21 ), and the fatty acid profiles of tif-1A KD being consistent with elevated activity of Δ9 desaturases [38] , [39] (Fig. 5b and Supplementary Fig. 8a ). These findings suggest that at least some of the lipidome remodeling events occurring in Pol I modulated animals are not causally linked to longevity, reemphasizing the specific role of TAG metabolism in Pol I-linked geroprotection. Fig. 6: TAG lipolysis mediates longevity effects of the differential Pol I activity. a , b Survival analysis of wild-type (N2 Bristol strain) nematodes exposed to control (Ctrl), rpoa-2 and atgl-1 RNAi, or simultaneously to rpoa-2 and atgl-1 RNAi ( a ) or Ctrl, ncl-1 and atgl-1 RNAi, or simultaneously to ncl-1 and atgl-1 RNAi ( b ). c Survival analysis of N2 and prx-5 (ku517) mutant nematodes exposed to Ctrl or rpoa-2 RNAi. d Survival analysis of wild-type worms exposed to Ctrl, rpoa-2 , acs-2 RNAi or double RNAi targeting rpoa-2 and acs-2 . Survival was scored daily, and n = 140 worms in all tests. Statistics were calculated using Mantel-Cox test. e Mitochondrial oxygen consumption rate (OCR) measured on AD12 in wild-type nematodes treated with Ctrl, tif-1A or ncl-1 RNAi. OCR was normalized to the number of worms and mean ± S.E.M. of n = 85 animals is shown. Statistical analysis was performed by using unpaired t -test on area under the curve values. ns = not significant, **** P < 0.0001, *** P < 0.001, ** P < 0.01, * P < 0.05. Representative results of 3 independent experiments are shown in all cases. All statistical tests used were two-sided, the exact P values and statistical analyses are reported in the Source Data file. f Schematic representation of the molecular mechanism connecting curbed Pol I activity with the attenuation of metabolic aging. The image was created with BioRender.com. Full size image We next tested if inhibition of atgl-1 affects mitochondrial stress in tif-1A and ncl-1 KDs. Interestingly, inactivation of atgl-1 reversed high levels of hsp-6p::GFP expression in ncl-1 RNAi-treated worms, while very low mito-stress levels of tif-1A KD nematodes were not further reduced by co-treatment with atgl-1 RNAi, suggesting that ATGL-1 activity might be already lowered in response to Pol I repression (Supplementary Fig. 15a, b ). These data reveal ATGL-1-dependent TAG lipolysis, which is likely elevated in ncl-1 KD and reduced in tif-1A KD animals, to be an instigator of mitochondrial stress. Notably, increased lipolysis of TAGs and the subsequently increased flux of fatty acids into mitochondria were recently linked to alterations in mito-homeostasis and elevated oxygen consumption rate (OCR) [57] . We next measured OCR levels in ncl-1 and tif-1A KDs at the age with the strongest difference in their TAG expenditure (AD12, Fig. 5a ), and found oxygen consumption to be elevated in ncl-1 RNAi-treated animals, while tif-1A KD worms showed diminished OCR levels (Fig. 6e ). As OCR is a contributor to reactive oxygen species (ROS) production and oxidative stress [58] , enhanced TAG lipolysis likely fuels the mitochondrial damage and the accelerated aging phenotype of NCL-1-depleted worms. Conversely, tif-1A KD animals exhibited reduced TAG turnover and lower OCR, presumably resulting in preservation of mitochondrial health and aging deceleration (Fig. 6f and Supplementary Fig. 16 ). However, as atgl-1 RNAi treatment abrogates life extension of tif-1A KD animals (Fig. 6a ), a basal level of TAG mobilization seems to be essential for health maintenance of tif-1A -depleted animals. This notion is supported by modestly increased mitochondrial stress levels of worms co-treated with tif-1A and atgl-1 RNAis (Supplementary Fig. 15a, b ). Finally, we found that depletion of SKN-1/Nrf2 not only abrogates longevity benefits of Pol I inhibition (Fig. 5g ), but also limits the accumulation of TAGs induced by rpoa-2 KD (Supplementary Fig. 14a ). This observation suggests that SKN-1 might be implicated in the regulation of TAG turnover downstream of rDNA transcription, which is consistent with its previously reported role in lipid catabolism [59] . However, future studies are required to systematically validate this hypothesis. Pol I-linked geroprotection is not restricted by age In light of recently uncovered age limitations of geroprotective interventions such as metformin and DR [13] , [14] , we used the rapidity of the rpoa-2 knockdown to explore at which stage in life attenuation of pre-rRNA synthesis is beneficial. First, we initiated the rpoa-2 RNAi treatment at AD0, AD6, or AD8, and measured rpoa-2 mRNA and pre-rRNA levels at AD10 (Fig. 7a–c ). Both parameters were affected stronger by RNAi administered earlier in life, presumably reflecting the longer exposure to the dsRNA-producing bacteria and the higher rate of their ingestion early in adulthood [35] (Fig. 7b , c). Based on these results, we assumed that the timeline of survival experiments ( ∼ 30 days) was sufficient for gene inactivation in all cases. Accordingly, the median lifespan was prolonged to a similar extent regardless of the stage in life when the rpoa-2 knockdown was started (Fig. 7d ), showing that initiating Pol I perturbation post-middle age is a robust pro-longevity intervention. Fig. 7: Curbing of Pol I activity promotes healthy longevity independently of age. a Schematic of the strategy for rpoa-2 inactivation at different ages and subsequent analysis of the animals. The image was created with BioRender.com. b , c RT-qPCR analysis of rpoa-2 mRNA ( b ) and pre-rRNA ( c ) levels at AD10 in nematodes treated with either control (Ctrl) RNAi or rpoa-2 RNAi from AD0, AD6 or AD8 onwards. Data are relative to Ctrl RNAi values and normalized to tgb-1 mRNA. Samples from 3 independent experiments with n = 60 animals per sample were analyzed, mean ± S.D. is shown. d Lifespan analysis of animals treated with Ctrl RNAi or with rpoa-2 RNAi from AD0, AD6 or AD8 onwards. n = 140 worms, survival was scored daily. Result is representative of 3 independent tests. e Locomotor performance tests (burrowing assays) at AD10 after Ctrl RNAi or rpoa-2 RNAi were administered as shown in ( a ). Percentage of animals that have reached the surface within indicated time is shown. Data are from 3 independent trials with n = 40 worms per group, mean ± S.D. values are shown. f Quantification of ‘Smurf’ animals showing intestinal leakage after RNAi treatments as indicated in ( a ). Percentage of worms with whole body staining from n = 40–50 worms per treatment is presented. Mean ± S.D. values from 3 independent trials are shown. P values were determined with an unpaired Student’s t -test ( b , c , f ) or Mantel-Cox test ( d , e ). ns = not significant, **** P < 0.0001, *** P < 0.001, ** P < 0.01, * P < 0.05. All statistical tests used were two-sided, the exact P values and statistical analyses are reported in the Source Data file. Full size image In nematodes, aging-associated tissue deterioration sets in shortly after the end of reproduction around AD6 [60] . To test whether RPOA-2 depletion starting at AD6 or later can improve healthspan, burrowing assays were performed at AD10 after nematodes were transferred to rpoa-2 RNAi at AD0, AD6, and AD8. Control worms were clearly outperformed by all three rpoa-2 RNAi-treated groups (Fig. 7e ). Similarly, Smurf assays showed that late-life RPOA-2 depletion improved intestinal integrity (Fig. 7f ). Thus, although lowering of Pol I activity throughout adulthood was most beneficial, its initiation late in life still efficiently decelerated tissue deterioration and improved health. Here, we uncovered that curtailment of pre-rRNA synthesis triggers multiple geroprotective adaptations in C. elegans , while elevation of rDNA activity confers an early advantage in fitness at the expense of premature aging. While previous reports of lifespan extension through reduced pre-rRNA and 5S rRNA synthesis focused on links to nucleolar size, nucleolar architecture and protein synthesis [7] , [8] , [61] , we have discovered a novel metabolic remodeling response that mediates pro-longevity effects of Pol I impairment. Our in-depth analyses demonstrated that curtailment of pre-rRNA synthesis attenuates metabolic aging and stabilizes energy turnover, providing an ATP surplus for healthy homeostasis. Importantly, we found a similar energy preservation effect upon depletion of the ribosomal protein RPS-15 previously linked to life span extension in C. elegans [30] . Notably, no energy saving was detected upon restriction of translation initiation or elongation. While we cannot rule out that the curtailment of protein synthesis is more effective when targeting ribosome biogenesis instead of translation, the former will additionally reduce cellular ATP consumption by blocking ribosome assembly and restricting pre-rRNA synthesis and processing [4] , [5] , [29] . In line with this notion, distinct longevity mechanisms triggered by ribosomal protein depletion and inhibition of translation have been reported [30] . We also found that immune, proteostasis, and oxidative stress responses with known dependency on DAF-16/FOXO activity [62] , [63] were not changed in tif-1A and ncl-1 inactivated animals. This finding corroborates observations of daf-16 being dispensable for the longevity extension by the depletion of ribosomal proteins, while it is required for the survival effects of translational repression [30] . Specifically, our data demonstrate that dampened Pol I activity preserves metabolic plasticity throughout life, as showcased by lowered mitochondrial stress at a young age and elevated late-life metformin resilience of worms with perturbed Pol I machinery. Concurrently, lowered Pol I activity triggers lipidome remodeling towards reduced abundance of damage-prone and lipotoxic phospholipids and fatty acids, with increased Pol I activity conferring the opposite effect on both mitochondrial stress and the lipidome. The most notable difference in lipidome profiles was the differential expenditure of cellular TAG storage, which was enhanced in ncl-1 KD and reduced in tif-1A KD during aging. Remarkably, in both cases, the changes in lifespan could be reversed by the depletion of the lipase ATGL-1, which initiates TAG catabolism [51] . ATGL-1 is activated during fasting to facilitate the extraction of energy from TAGs [53] but at the same time, its activity is dampened during dauer diapause to ration TAG usage during the exceptional longevity of the dauer larvae [52] . It is thus feasible that ATGL-1 activity is modulated by changes in energy levels downstream of differential Pol I output. In this context, tif-1A and rpoa-2 KDs exhibited increased TAG levels, indicating slower TAG expenditure similar to the dynamics observed in dauer larvae, while TAG levels in ncl-1 KD suggest accelerated TAG catabolism. Such differences in TAG mobilization are likely influencing the levels of FAs that are released from TAGs and further processed by mitochondria dictating oxygen consumption rate (OCR) and expression of mitochondrial homeostasis genes [57] . Consistently, we found OCR to be elevated in ncl-1 KD nematodes, while it was lowered in tif-1A KD animals. We also found that depletion of ATGL-1 reduces mitochondrial stress levels in the background of ncl-1 KD. Given the connection between OCR and ROS production by the electron transport chain [58] , our findings suggest that curbing of Pol I activity preserves mitochondrial health by attenuating TAG catabolism and thereby restricting OCR. Conversely, boosted rDNA transcription accelerates TAG turnover, in turn promoting oxygen consumption, damage of mitochondria, and premature aging (Fig. 6f and Supplementary Fig. 16 ). The premature demise of ncl-1 KD worms delivers a note of caution for recreational self-treatments that activate TOR (e.g. high protein diets) and thereby boost Pol I activity. Such treatments do promote rapid improvements in fitness as seen in ncl-1 deficient nematodes, but may accelerate metabolic aging in the long-term. Despite the diversity of observed lipidome changes, only TAG lipolysis was critical for the geroprotective effects of lowered rDNA transcription. It is thus plausible that at least some of the detected lipidome adaptations occurred as a result of altered TAG turnover. In line with this hypothesis, TAG cycling was linked to dynamic changes in the cellular FA repertoire [64] , and increased accumulation of TAGs in lipid droplets was associated with the geroprotective lipidome remodeling in nematodes exposed to high levels of MUFA-lipids [65] . Importantly, we show that curbing of Pol I activity retains its geroprotective capacity also late in life, unlike DR and metformin treatment, which indirectly regulate Pol I [10] , [11] , [12] . It is conceivable that inhibition of pre-rRNA synthesis allows bypassing the adaptive failures that limit late life efficacy of metformin and DR [13] , [14] by acting directly on one of their prominent downstream targets. In addition, we provide evidence of metabolic stress protection by pharmacological Pol I inhibition in human primary cells. While our results raise hope for a new longevity treatment, interference with pre-rRNA synthesis in vivo would need to be carefully tuned. Pol I perturbation early in life comes with the risk of impaired development and growth retardation as seen in congenital diseases termed ribosomopathies [66] . Accordingly, our data suggest that initiating moderate Pol I inhibition in late life would bypass the potential developmental trade-offs and instead counteract the aberrant increase in rRNA production that has been reported in normal and pre-mature human aging [67] . C. elegans strains and maintenance C. elegans strains were cultured under standard conditions as described in ‘Wormbook’ [68] . Age-synchronization of worms by bleaching was performed as previously described [69] . Experimental temperatures for all figures are summarized in Supplementary Data 23 . The C. elegans wild isolate (Bristol N2), ife-2(ok306) mutant (KX15), atfs-1(gk3094) mutant (VC3201), pink-1(tm1779) mutant (BR4006, without transgene), skn-1(zj15) mutant (QV225), prx-5(ku517) mutant (MH5239), myo-3p::gfpmt (zcls14) expressing strain (SJ4103), hsp-6p::GFP expressing strain (SJ4100) and FIB-1::GFP expressing strain (COP262) were obtained from the NIH funded Caenorhabditis Genetics Centre (CGC). E. coli OP50 and HT115 strains were obtained from CGC. The tif-1A overexpressing strain C0P2239 (genotype: 3p::3xTy1::C36E8.1::tbb-2u in ttTi5605, unc-119( + ) ) II; unc 119(ed3) III) was generated by InVivo Biosystems using the MosSCI method [70] . RNA interference experiments RNAi experiments were prepared as described elsewhere [71] using bacterial strains from the Ahringer RNAi feeding library (Source BioScience Ltd.). ncl-1 and tif-1A knockdown was achieved by feeding the worms with bacteria producing the corresponding dsRNA for two generations at 15 °C. To achieve rpoa-2 and atgl-1 knockdown, L4 larvae or adult worms of the indicated ages were transferred on the dsRNA-producing bacteria and kept throughout the experiment at 20 °C, unless stated otherwise. RNAi treatment durations for all figures are summarized in Supplementary Data 23 . Lifespan analysis in C. elegans For lifespan analysis without RNAi treatment, age-synchronized worms were reared on nematode growth medium (NGM) agar with E. coli OP50 at 20 °C. If RNAi treatment was conducted during lifespan analysis, worms were kept at 15 or 20 °C as indicated in Supplementary Data 23 , and NGM agar contained 1.5 mM Isopropyl-β-D-thiogalactopyranosid (IPTG, Sigma-Aldrich, I6758) and was seeded with a dsRNA-producing E. coli HT115(DE3) strain [72] . For each assay condition, two 60 mm plates with initially 70 worms each were used. Animals were transferred to fresh plates every second day during the reproductive phase and every 4 days in the post-reproductive phase. Worms were scored daily, and dead worms were removed. For lifespan analysis in the presence of drugs, cycloheximide (Sigma-Aldrich, 01810), Carbonyl cyanide-p-trifluoromethoxyphenylhydrazone (FCCP) (Cayman chemical, Cay15218-10) and metformin (M2009, TCI) were added to the agar to a final concentration of 10, 20, 25 µM and 50 mM, respectively. DMSO (Sigma-Aldrich, D2438) was used as a solvent for FCCP at a final concentration of 0.05%. Burrowing assay The burrowing assay was performed as previously described [17] . Briefly, 50 µl of a 26% pluronic F-127 gel (Sigma-Aldrich, P2443) (w/w, dissolved in H2O) were solidified at the bottom of a 35 mm plate and 40-45 worms were placed on top. Animals were overlayed with 4 ml of the same gel and after hardening, 20 µl of concentrated E. coli OP50 suspension (100 mg/ml) was added as a chemoattractant on the surface. Animals reaching the surface were recorded every 15 or 30 min for 2 or 3 h. Three plates per condition were used in each experiment. Smurf assay Smurf assay was performed following a previously described method [19] . In brief, nematodes were incubated in a E. coli OP50 liquid culture containing 5% Brilliant Blue FCF (Sigma-Aldrich, 80717) for 3 h at 18 °C. Afterward, worms exhibiting blue staining outside of the intestine (Smurf) were scored using Zeiss Axio Zoom.V16 microscope at the magnification of ×25. Nucleolar and worm size measurement FIB-1::GFP expressing nematodes were washed with M9 buffer and transferred to poly-L-lysine-coated microscopy slides (Sigma-Aldrich, P5899). M9 buffer was removed and worms were fixed in 10 μl ethanol. After evaporation of the ethanol, fixation was repeated and slides were mounted with mounting media containing 4´,6-diamidino-2-phenylindole (DAPI). The specimens were imaged on Zeiss Axiovert 200 ApoTome (Carl Zeiss AG). Nuclei (DAPI staining, Abcam PLC, ab104139), and nucleoli (FIB-1::GFP staining) in individual cells were contoured and the corresponding areas were quantified using the ZEISS ZEN Imaging Software. For determining worm size, bright field images were recorded, and the areas of animals were measured with the same software. Gene expression analysis For extraction of total RNA, worms were washed twice in M9 buffer, resuspended in TRI reagent (Sigma-Aldrich, T9424), and lysed with a Precellys tissue homogenizer (Bertin Technologies SAS). BJ cells were harvested and directly lysed in TRIzol (Thermo Fisher Scientific/Invitrogen, 15596018). Total RNA was isolated and 1 μg was treated with DNase I (Sigma-Aldrich/Merck, AMPD1-1KT) in the presence of 0.25 μl RNase inhibitor (RiboLock, Thermo Fisher Scientific, EO0384) for 20 min at room temperature. cDNA was synthesized with random hexamers (Roche, 11034731001) using SuperScript IV Reverse Transcriptase (Thermo Fisher Scientific, 18091200 and 18090050) according to the manufacturer’s recommendation. The cDNA was amplified in a two-step quantitative PCR (qPCR) using SYBR Green Maxima SYBR Green/ROX 2X qPCR Master Mix (Thermo Fisher Scientific, K0222) following the manufacturer’s instructions. QuantStudio™ 3 real-time-PCR instrument (Applied Biosystems, Foster City, USA) was used. Primer sequences are provided in Supplementary Data 22 . ATP measurements ATP content was measured as previously described [73] with minor modifications. Briefly, 50 worms were washed twice and resuspended in 1 ml M9 buffer, followed by snap-freezing and boiling for 10 min. After sonication in a Bioruptor Plus (Diagenode) (10 cycles, 1 min on, 30 s off), lysates were cleared by centrifugation at 15,300 × g at 4 °C for 10 min. To determine relative ATP levels, the “ATP Bioluminescence Assay Kit HS II” (Roche, 11699709001) was used according to the manufacturer’s instructions, and measurements were carried out in a Mithras LB 940 microplate reader (Berthold). Data were normalized to the protein concentrations of the samples as measured by absorbance at 280 nm (A280) in a NanoDrop photometer (Thermo Fisher Scientific). Western blot analysis 700 worms were lysed as for ATP measurements by snap freezing, boiling, and sonication. 30–50 µg of total protein were resolved by 10% polyacrylamide gel electrophoresis (PAGE). Proteins were transferred to a nitrocellulose membrane by semi-dry blotting on a Trans-Blot Turbo Transfer System (Bio-Rad Laboratories). Immunodetection was performed with primary anti-Ty1 (Diagenode, C15200054, Lot 007) or anti-tubulin (Sigma-Aldrich, clone DM1A, T6199) antibodies, followed by probing with a horseradish peroxidase-conjugated anti-mouse antibody (Dianova, DkxMu-003-FHRPX, Lot 67-83-071919). Antibody dilutions were 1:5000 for primary, and 1:10,000 for secondary antibodies. Blots were developed with a SuperSignal west pico PLUS chemiluminescent substrate (Thermo Fisher Scientific, 34580) and imaged on a Fusion Solo 4S system (Vilber Lourmat). Sample preparation for proteomics Proteomics analysis was conducted as previously described [14] . Briefly, 700 worms were harvested for each sample and transferred to Precellys CKMix Lysing Kits tubes containing 1.4 mm and 2.8 mm ceramic beads (Bertin Technologies). Samples were adjusted with 25 µl 10 x lysis buffer (final concentrations 4% SDS, 100 mM HEPES, pH 8.5, 50 mM DTT) and homogenized using a Precellys 24 tissue homogenizer (Bertin Technologies) for 3 cycles (6000 mixes for 20 s followed by 30 s pause). Beads were sedimented and supernatants were sonicated (Bioruptor Plus, Diagenode) for 10 cycles (30 s ON/60 s OFF) at 20 °C, followed by boiling at 95 °C for 5 min. Reduction was followed by alkylation with 20 mM iodoacetamide (IAA, final concentration 15 mM) for 30 min at room temperature in the dark. Protein amounts were estimated by SDS-PAGE and Coomassie blue staining of an aliquot of each sample by comparing the staining intensity to a quantified standard cell extract prepared from mouse embryonic fibroblasts. 30 µg protein was further processed for digestion. Proteins were precipitated with four volumes of ice-cold acetone overnight at −20 °C and sedimented by centrifugation at 20,800 × g for 30 min at 4 °C, followed by two washes with 300 µL ice-cold 80% (v/v) acetone in water. Protein pellets were air-dried and resuspended by sonication in 25 µl of digestion buffer (1 M Guanidine, 100 mM HEPES, pH 8). LysC (Wako) was added at 1:100 (w/w) enzyme to protein ratio and digestion proceeded for 4 h at 37 °C. Samples were then diluted with one volume of MilliQ water and trypsin (Promega) was added at a 1:100 (w/w) enzyme:protein ratio. After digestion overnight at 37 °C, trifluoroacetic acid was added to a final concentration of 10% (v/v), and samples were desalted with Waters Oasis® HLB µElution Plate 30 µm (Waters Corporation) under a soft vacuum following the manufacturer’s instruction. Samples were dried down using a speed vacuum centrifuge (Eppendorf Concentrator Plus) and redissolved at a concentration of 1 µg/µl peptides in reconstitution buffer (5% (v/v) acetonitrile, 0.1% (v/v) formic acid in MilliQ water). LC-MS/MS proteomics Reconstituted peptides were spiked with the retention time normalization iRT kit (Biognosys) and separated in trap/elute mode using the nanoAcquity MClass Ultra-High Performance Liquid Chromatography system (Waters, Waters Corporation) equipped with a trapping (nanoAcquity Symmetry C18, 5 μm, 180  μm × 20 mm) and an analytical column (nanoAcquity BEH C18, 1.7 μm, 75 μm × 250 mm). The outlet of the analytical column was coupled directly to an Orbitrap Q exactive HF-X mass spectrometer (Thermo Fisher Scientific) using the Proxeon nanospray source. Solvent A was water and 0.1% formic acid, and solvent B was acetonitrile and 0.1% formic acid. The samples ( ∼ 1 μg) were loaded with a constant flow of solvent A at 5 μl/min onto the trapping column. Trapping time was 6 min. Peptides were eluted via the analytical column with a constant flow of 0.3 μl/min. During the elution step, the percentage of solvent B increased in a nonlinear fashion from 0–40% in 120 min. Total run time was 145 min. The peptides were introduced into the mass spectrometer via a Pico-Tip Emitter 360-μm outer diameter × 20-μm inner diameter, 10-μm tip (New Objective) heated at 300 °C, and a spray voltage of 2.2 kV was applied. The capillary temperature was set at 300 °C. The radiofrequency ion funnel was set to 40%. For DIA data acquisition, full-scan mass spectrometry (MS) spectra with mass range 350–1650 m/z were acquired in profile mode in the Orbitrap with a resolution of 120,000 FWHM. The default charge state was set to 3+. The filling time was set at a maximum of 60 ms with a limitation of 3 × 106 ions. DIA scans were acquired with 40 mass window segments of different widths across the MS1 mass range. Higher collisional dissociation fragmentation (stepped normalized collision energy; 25.5, 27, and 30%) was applied and MS/MS spectra were acquired with a resolution of 30,000 FWHM with a fixed first mass of 200 m/z after accumulation of 3 × 106 ions or after filling time of 35 ms (whichever occurred first). Data were acquired in profile mode. For data acquisition and processing of the raw data, Xcalibur 4.0 (Thermo Fisher) and Tune version 2.9 were used. Proteomics data analysis DIA raw data were analyzed using the directDIA pipeline in Spectronaut (v.13, Biognosysis AG). The data were searched against UniProt and a species-specific ( C. elegans , 26.677 entries) Swissprot database. The data were searched with the following modifications: Carbamidomethyl (C) (Fixed) and Oxidation (M)/ Acetyl (Protein N-term) (Variable). A maximum of 2 missed cleavages for trypsin was allowed. The identifications were filtered to satisfy FDR of 1% on peptide and protein levels. Relative quantification was performed in Spectronaut for each paired and unpaired comparison using the replicate samples from each condition. The data (candidate table) and data reports (protein quantities) were then exported and further data analyses and visualization were performed with Rstudio using in-house pipelines and scripts [74] . Differently regulated proteins were analyzed for biological functions using WormCat [23] . Lipidomics For each lipidomics analysis, 700–800 age-synchronized worms were washed with M9 medium and shock-frozen in 100 µl medium. Liquid-liquid-extraction of lipids and subsequent targeted lipidomics was performed as reported [14] , [75] . In brief, glycerophospholipids (i.e., phosphatidylcholine, phosphatidylethanolamine, phosphatidylinositol, phosphatidylserine), glycerolipids (i.e., TAG) and free fatty acids were separated on an ACQUITY UPLC system (Waters) with a reversed-phase column (ACQUITY UPLC BEH C8; 1.7 μm, 2.1 × 100 mm; Waters) using previously established settings [14] . The LC system was coupled to a QTRAP 5500 mass spectrometer (Sciex) equipped with an electrospray ionization source, which was operated by Analyst 1.6.2 (Sciex). Lipids were measured by multiple or selected reaction monitoring in the negative (glycerophospholipids, free fatty acids) or positive ion mode (triacylglycerols) [14] , and extracted chromatograms were processed using Analyst 1.6.3 (Sciex). The absolute abundance of different lipid classes represents the summarized signal intensities of all analyzed lipid species of an indicated lipid class (for example, all analyzed PCs), which are normalized to the internal standard 1,2-dimyristoyl-sn-glycero-3-phosphocholine (DMPC; 850345P, Avanti Polar Lipids) as well as the number of worms. Proportions of individual lipids or lipid scores (e.g., TAGs with a unique total fatty acid chain length) were calculated as ratio of signal intensities (e.g., from individual TAG species) to the summarized total signal intensity of a given lipid class (e.g., TAGs). Cell culture For MTT assays, BJ human skin fibroblasts (ATCC, #CRL-2522) were cultured in an incubator with a humidified atmosphere at 37 °C and 5% CO 2 as previously described [14] . Briefly, cells were grown in complete Dulbecco’s modified eagle’s medium (DMEM) (high glucose media, Sigma-Aldrich/Merck, D6429) supplemented with 10% of fetal bovine serum (FBS) (Sigma-Aldrich/Merck, F7524). Cells were seeded in 96 flat well plates at a density of 30,000 cells per well and incubated overnight prior to treatment. For the 24h-long pre-treatment with Pol I inhibitors or DMSO (Sigma Aldrich/Merck, D2438), complete DMEM was used. For metformin treatment, the media was replaced with glucose-free DMEM (Thermo Fischer Scientific, A1443001) supplemented with 10% FBS only. DMSO was used as solvent for the inhibitors at a final concentration of 0.01%. For gene expression analysis, cells were maintained in StableCell™ DMEM (Sigma-Aldrich/Merck, D0819) high glucose, supplemented with 10% FBS (Capricorn Scientific, FBS-11A), 100 units/mL penicillin and 0.1 mg/mL streptomycin (Sigma-Aldrich /Merck, P4333). Cells were seeded and incubated overnight prior to the treatment with Pol I inhibitors or DMSO (Sima-Aldrich/Merck, Cat# D2650), which lasted 24 h. Mitochondrial activity assay Filtered MTT solution (Sigma Aldrich/Merck, M5655) was added to cell cultures at a final concentration of 1 mg/mL. Plates were incubated for 3 h (37 °C, 5% CO 2 ) with light protection followed by media replacement with the MTT solubilization agent (0.1 N HCL, Roth X942.1 in absolute isopropanol, Roth 6752.3). Specific MTT absorbance was measured at 570 nm and background - at 690 nm, using a plate-reading spectrophotometer (Infinite M1000 Pro, Tecan). Metformin (M2009, TCI), BMH-21 (SML1183, Merck) and CX-5461 (HY-13323A, MCE) were used for treatment. Assessment of mitochondrial stress and mitochondrial morphology hsp-6p::GFP worms were age-synchronized and fed with empty vector (Ctrl), mip-1 RNAi, tif-1A RNAi, or ncl-1 RNAi bacteria (Ahringer library) from L4 stage of the previous generation. F1 adults were bleached and F2 progeny were used for the imaging on adulthood day 2 (AD2) using AxioZoom_V16 microscope (Zeiss) at ×90 magnification. Fluorescence was measured as the mean intensity value obtained from the GFP channel for each worm using the Zen blue (2.6 edition) software. For morphology tests, myo-3p::gfpmt expressing worms were fed with empty vector (Ctrl) RNAi from L1 stage and transferred to Ctrl, rpoa-2 RNAi, or ncl-1 RNAi at L4 stage, and % of tubular, intermediate, fragmented and very fragmented mitochondria was assessed on day 2 of adulthood as previously described [14] . Assessment of mitochondrial OCR by Seahorse Wild-type nematodes were age-synchronized and fed with empty vector (Ctrl), tif-1A RNAi or ncl-1 RNAi bacteria (Ahringer library) from L4 stage of the F0 generation at 20 °C. F1 adults were bleached and F2 progeny were shifted to 15 °C at L4 stage and later used for the OCR measurement on day 12 of adulthood. Worms were rinsed off the plates and washed three times with 1X M9 buffer to remove traces of bacteria. Worms were then suspended in 1 ml EPA water and transferred to individual wells of a 96 well plate (20–30 worms/well). FCCP (Cayman chemical, Cay15218-10) and Rotenone (Sigma Aldrich/Merck, R8875) were dissolved in DMSO (Sigma Aldrich/Merck D2438) prior to assessment and diluted in EPA water to obtain the working concentration of 200 µM and 50 µM, respectively. 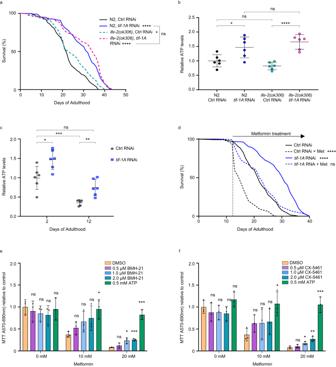Fig. 4: Pol I inhibition decelerates metabolic aging. aSurvival analysis ofC. eleganswild-type (N2 Bristol) andife-2mutant strains treated with control (Ctrl) RNAi ortif-1ARNAi,n= 140 worms.bComparison of ATP pools at AD2 between wild-type (N2) andife-2mutant worms treated with Ctrl RNAi ortif-1ARNAi. ATP levels were measured in a bioluminescence assay and normalized to total protein content. Values are shown relative to N2 Ctrl RNAi. Data are from 6 independent experiments withn= 50 worms in each sample. Mean ± S.D. values are shown.cComparison of ATP pools at AD2 and AD12 between worms treated with Ctrl RNAi ortif-1ARNAi. ATP measurement was conducted as inb, and values are relative to Ctrl RNAi on AD12. Mean ± S.D. values of 6 independent experiments withn= 50 worms are shown.dSurvival analysis of worms exposed to Ctrl RNAi ortif-1ARNAi and, from AD12 onwards, to 50 mM metformin (Met),n= 140 animals. A representative result of four independent experiments is shown. Foraandd, survival was scored daily andPvalues were determined using the Mantel-Cox test. Forbandc, a Student’s unpairedt-test was used for statistics.e,fBJ primary human skin fibroblasts were treated with indicated doses of metformin in the absence (DMSO) or presence of the indicated concentrations of ATP (positive survival control) or the Pol I inhibitors BMH-21 (e) and CX-5461 (f). Mitochondrial activity was assessed by MTT assay, and an unpaired Student’st-test was used to computePvalues, comparing each co-treatment to the respective DMSO + Metformin control condition, data represent mean ± S.D of 3 independent experiments. ns = not significant, ****P< 0.0001, ***P< 0.001, **P< 0.01, *P< 0.05. All statistical tests used were two-sided, the exactPvalues and statistical analyses are reported in the Source Data file. The assay was performed in 96-well plate in Agilent Seahorse XF Pro analyser. 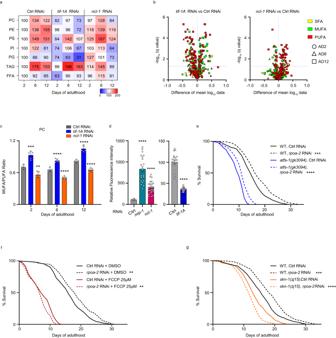Fig. 5: Pol I activity affects the lipidome and mitochondria. aLipid abundance in control (Ctrl) RNAi,tif-1ARNAi andncl-1RNAi animals at different ages, normalized to the internal standard and animal number (n= 700). Values were computed from absolute intensities; mean of 5 biological replicates expressed as % of Ctrl RNAi treatment at AD2 is shown in each case (see Supplementary Data12for raw data). PC phosphatidylcholine, PE phosphatidylethanolamine, PS phosphatidylserine, PI phosphatidylinositol, PG phosphatidylglycerol, TAG triacylglycerol, FFA free fatty acid.bVolcano plots of lipid species separated by age (AD 2, 6, 12) and fatty acid desaturation. SFA saturated fatty acid, MUFA monounsaturated fatty acid, PUFA polyunsaturated fatty acid. Horizontal axis subtracts Ctrl RNAi mean log10values from respectivetif-1ARNAi (left panel) orncl-1RNAi (right panel) values for each lipid, with statistics performed by multiple unpairedt-test on log-transformed mean values using a two-stage linear step-up procedure by Benjamini, Krieger and Yekutieli, FDR = 5%, data are from 5 biological replicates withn= 700 worms each. Calculations (from relative intensities) are shown in Supplementary Data13–15.cRatio of MUFAs to PUFAs in PCs at indicated age upon treatment with Ctrl RNAi,tif-1ARNAi orncl-1RNAi. Mean ± S.D. values from 5 replicates each withn= 700 worms are shown. Calculations (from relative intensities) are shown in Supplementary Data19.dFluorescence measurements in nematodes expressinghsp-6p::GFPfollowing exposure to Ctrl,mip-1,ncl-1ortif-1ARNAi.mip-1RNAi served as a positive mito-stress control.n= 20-25 worms per condition. Representative result of 3 independent trials. Forcandd, Student’s unpairedt-test comparedncl-1andtif-1ARNAi effects to the age-matched Ctrl RNAi baseline.e–gSurvival analysis of wild-type (N2 Bristol strain) andatfs-1 (gk3094)mutant nematodes (e), or N2 worms treated from AD1 onwards with the vehicle DMSO or 25 µM FCCP (f), or N2 andskn-1 (zj15)mutant nematodes (g), exposed to Ctrl orrpoa-2RNAi, survival was scored daily. Representative results of three independent experiments,n= 140 worms, statistics assessed by Mantel-Cox test. ns = not significant, ****P< 0.0001, ***P< 0.001, **P< 0.01, *P< 0.05. All statistical tests used were two-sided, the exactPvalues and statistical analyses are reported in the Source Data file. Data was normalized to the number of worms. Statistical analysis Experiments were performed in biological replicates as stated in the figure legends. Statistical analysis was performed with Prism 8 (Graphapd Software Inc.). All bar graphs show the mean values with error bars (±S.D. or ±S.E.M as indicated in the legends). 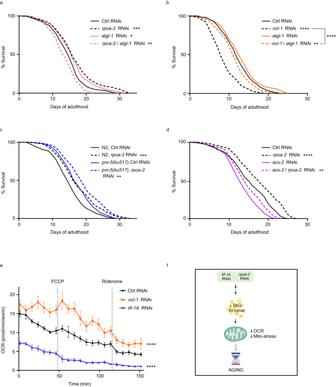Fig. 6: TAG lipolysis mediates longevity effects of the differential Pol I activity. a,bSurvival analysis of wild-type (N2 Bristol strain) nematodes exposed to control (Ctrl),rpoa-2andatgl-1RNAi, or simultaneously torpoa-2andatgl-1RNAi (a) or Ctrl,ncl-1andatgl-1RNAi, or simultaneously toncl-1andatgl-1RNAi (b).cSurvival analysis of N2 andprx-5 (ku517)mutant nematodes exposed to Ctrl orrpoa-2RNAi.dSurvival analysis of wild-type worms exposed to Ctrl,rpoa-2,acs-2RNAi or double RNAi targetingrpoa-2andacs-2. Survival was scored daily, andn= 140 worms in all tests. Statistics were calculated using Mantel-Cox test.eMitochondrial oxygen consumption rate (OCR) measured on AD12 in wild-type nematodes treated with Ctrl,tif-1Aorncl-1RNAi. OCR was normalized to the number of worms and mean ± S.E.M. ofn= 85 animals is shown. Statistical analysis was performed by using unpairedt-test on area under the curve values. ns = not significant, ****P< 0.0001, ***P< 0.001, **P< 0.01, *P< 0.05. Representative results of 3 independent experiments are shown in all cases. All statistical tests used were two-sided, the exactPvalues and statistical analyses are reported in the Source Data file.fSchematic representation of the molecular mechanism connecting curbed Pol I activity with the attenuation of metabolic aging. The image was created with BioRender.com. 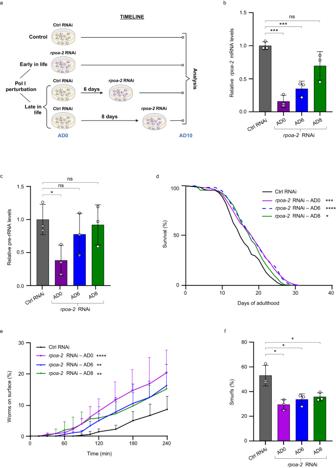Fig. 7: Curbing of Pol I activity promotes healthy longevity independently of age. aSchematic of the strategy forrpoa-2inactivation at different ages and subsequent analysis of the animals. The image was created with BioRender.com.b,cRT-qPCR analysis ofrpoa-2mRNA (b) and pre-rRNA (c) levels at AD10 in nematodes treated with either control (Ctrl) RNAi orrpoa-2RNAi from AD0, AD6 or AD8 onwards. Data are relative to Ctrl RNAi values and normalized totgb-1mRNA. Samples from 3 independent experiments withn= 60 animals per sample were analyzed, mean ± S.D. is shown.dLifespan analysis of animals treated with Ctrl RNAi or withrpoa-2RNAi from AD0, AD6 or AD8 onwards.n= 140 worms, survival was scored daily. Result is representative of 3 independent tests.eLocomotor performance tests (burrowing assays) at AD10 after Ctrl RNAi orrpoa-2RNAi were administered as shown in (a). Percentage of animals that have reached the surface within indicated time is shown. Data are from 3 independent trials withn= 40 worms per group, mean ± S.D. values are shown.fQuantification of ‘Smurf’ animals showing intestinal leakage after RNAi treatments as indicated in (a). Percentage of worms with whole body staining fromn= 40–50 worms per treatment is presented. Mean ± S.D. values from 3 independent trials are shown.Pvalues were determined with an unpaired Student’st-test (b,c,f) or Mantel-Cox test (d,e). ns = not significant, ****P< 0.0001, ***P< 0.001, **P< 0.01, *P< 0.05. All statistical tests used were two-sided, the exactPvalues and statistical analyses are reported in the Source Data file. For statistics, significance was determined at P < 0.05. The appropriate statistical test was chosen for each experiment as indicated in the figure legends and the Source Data file. Reporting summary Further information on research design is available in the Nature Portfolio Reporting Summary linked to this article.